The RNA helicase FRH is an ATP-dependent regulator of CK1a in the circadian clock ofNeurospora crassa The Neurospora clock protein FRQ forms a complex with casein kinase 1a (CK1a) and FRH, a DEAD box-containing RNA helicase with a clock-independent essential function in RNA metabolism. In the course of a circadian period, FRQ is progressively hyperphosphorylated and eventually degraded. Timed hyperphosphorylation of FRQ is crucial for timekeeping of the clock. Here we show that the ATPase activity of FRH attenuates the kinetics of CK1a-mediated hyperphosphorylation of FRQ. Hyperphosphorylation of FRQ is strictly dependent on site-specific recruitment of a CK1a molecule that is activated upon binding. The FRH ATPase cycle regulates the access of CK1a to phosphorylation sites in FRQ in cis , suggesting that FRH is an ATP-dependent remodelling factor acting on the protein complex. We show that the affinity of CK1a for FRQ decreases with increasing FRQ phosphorylation, suggesting functional inactivation of FRQ in the negative feedback loop of the circadian clock before and independent of its degradation. Circadian clocks are cell-autonomous molecular timing devices that rhythmically organize physiology and behaviour in a daily fashion. An essential aspect of time measurement on the molecular level in eukaryotes is the slowly progressing hyperphosphorylation by casein kinase 1 (CK1) of clock proteins acting in negative feedback loops of the core circadian oscillators [1] , [2] , [3] . Hyperphosphorylation of PERIOD proteins in mammals and flies and FREQUENCY (FRQ) in Neurospora strongly correlates with circadian timekeeping, but molecular mechanisms governing the slow yet precise phosphorylation kinetics of these proteins are poorly understood. In the course of a day, the Neurospora clock protein FRQ is progressively phosphorylated at ~100 sites [4] , [5] . FRQ interacts with CK1a [6] and forms a tight complex with FRQ-interacting RNA helicase (FRH), an essential DEAD box-containing RNA helicase [7] . DEAD box-containing RNA helicases comprise a large superfamily of ATPases whose functions are largely unknown [8] , [9] . Mtr4p, the Saccharomyces cerevisiae orthologue of FRH, is a component of the TRAMP complex and regulates RNA metabolism in cooperation with the nuclear exosome [10] , [11] , [12] , [13] . FRH is essential for the viability of Neurospora owing to its function in RNA metabolism [14] . In addition, FRH has been implicated in a variety of non-essential, clock-related functions: FRH is crucial for cytoplasmic localization and turnover of FRQ [15] , [16] , and also for the interaction of FRQ with the circadian transcription activator White Collar Complex (WCC) [15] , [17] . Furthermore, it was reported that FRH mediates turnover of frq RNA by committing the messenger for degradation by the exosome [14] . However, molecular mechanisms underlying these functions are not known. Recently, it has been suggested that the ATPase of FRH is not required for its function in the clock [18] . This conclusion was based on the assumption that dimeric FRQ interacts with only one molecule of FRH, as in the genetic background used the interaction of a FRQ dimer with two molecules of FRH could lead to cross-complementation by two functionally distinct FRH alleles present in the same complex [18] . Here we analysed the functional interaction of FRQ with FRH and CK1a in Neurospora , in a heterologous system in vivo and in a cell-free system with recombinant components. Our data demonstrate that the native FRQ–FRH complex (FFC) contains two FRH and two FRQ molecules. We show that the ATPase of FRH regulates the kinetics of hyperphosphorylation of FRQ by bound CK1a. Characterization of the FFC The polypeptide chains of FRQ and FRH have predicted molecular masses ( M r ) of 108 and 125 kDa, respectively. We analysed the interaction of FRQ with FRH and the stoichiometry of the components by gel filtration. The native FFC had an apparent M r of ~670 kDa. Although all FRQ is bound to FRH [7] , only ~15% of FRH were in complex with FRQ ( Fig. 1a and Supplementary Fig. 1a ). The fraction of FRH that is not associated with FRQ may serve non-circadian functions that are essential for the viability of Neurospora [7] . In constant darkness, when FRQ was rhythmically expressed, FRH levels remained constant ( Supplementary Fig. 1b ), indicating that the circadian clock does not control its expression level. 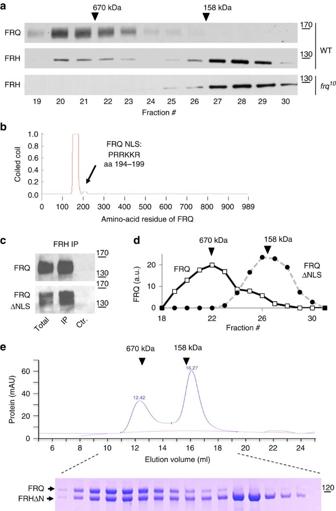Figure 1: Composition of the FFC. (a) Gel filtration analysis (Superose 6) of FRQ (108 kDa) and FRH (125 kDa) from wild-type (WT) andfrq10strains. The elution of molecular mass standards is indicated. (b) Prediction of coiled-coils (Expasy) in FRQ (989 amino acid residues). Dimerization/oligomerization of FRQ is dependent on the coiled-coil domain19. The location and composition of the NLS are indicated. (c) FRQΔNLS forms a stable complex with FRH. FRH fromWTandfrqΔNLS strains was immunoprecipitated with affinity-purified antibodies. Western blots were decorated with FRQ antibody to detect co-immunoprecipitation. (d) FRQΔNLS20does not form oligomeric complexes. Gel filtration (Superose 6) analysis of native protein extracts of light-grownWTandfrqΔNLSstrains. Densitometric quantification of western blots (Supplementary Fig. 1c) showing the elution profiles of FRQ and FRQΔNLS. (e)In vitroreconstitution of the FFC. Recombinant FRQ and FRHΔN (Supplementary Fig. 1d) form a ~670-kDa assembly with approximately 1:1 stoichiometry. Gel filtration (Superose 6) and SDS-PAGE analysis of the elution profiles of FRQ and FRHΔN are shown. Figure 1: Composition of the FFC. ( a ) Gel filtration analysis (Superose 6) of FRQ (108 kDa) and FRH (125 kDa) from wild-type ( WT ) and frq 10 strains. The elution of molecular mass standards is indicated. ( b ) Prediction of coiled-coils (Expasy) in FRQ (989 amino acid residues). Dimerization/oligomerization of FRQ is dependent on the coiled-coil domain [19] . The location and composition of the NLS are indicated. ( c ) FRQΔNLS forms a stable complex with FRH. FRH from WT and frq ΔNLS strains was immunoprecipitated with affinity-purified antibodies. Western blots were decorated with FRQ antibody to detect co-immunoprecipitation. ( d ) FRQΔNLS [20] does not form oligomeric complexes. Gel filtration (Superose 6) analysis of native protein extracts of light-grown WT and frqΔNLS strains. Densitometric quantification of western blots ( Supplementary Fig. 1c ) showing the elution profiles of FRQ and FRQΔNLS. ( e ) In vitro reconstitution of the FFC. Recombinant FRQ and FRHΔN ( Supplementary Fig. 1d ) form a ~670-kDa assembly with approximately 1:1 stoichiometry. Gel filtration (Superose 6) and SDS-PAGE analysis of the elution profiles of FRQ and FRHΔN are shown. Full size image FRQ forms a dimer or oligomer via its N-terminal coiled-coil domain [19] . We found that deletion of the nuclear localization signal (NLS) of FRQ [20] that is located next to the coiled-coil domain ( Fig. 1b ) did not affect its interaction with FRH but compromised oligomerization of FRQΔNLS (deletion of residues 194–199): Thus, FRH co-immunoprecipitated with FRQΔNLS ( Fig. 1c ) and the complex had a M r of ~250 kDa ( Fig. 1d and Supplementary Fig. 1c ), consistent with an assembly of one molecule FRQΔNLS with one molecule FRH. Accordingly, the wild-type ( WT ) complex should also contain equimolar amounts of FRQ and FRH. As FRQ is a dimer (or oligomer), the FFC (~670 kDa) should contain at least two molecules of FRQ and two molecules of FRH. To further address the stoichiometry of the FFC, we expressed FRQ, FRH and an N-terminally truncated FRH (FRHΔN) in Escherichia coli and purified the recombinant proteins ( Supplementary Fig. 1d ). FRQ formed a tight complex with FRHΔN (used for better separation from FRQ by SDS-PAGE), demonstrating that complex formation does not require ATP binding or hydrolysis by FRHΔN ( Fig. 1e ). The complex between FRQ and FRHΔN eluted from a gel filtration with an apparent M r >670 kDa was similar to the native Neurospora FFC. The complex between FRQ and FRHΔN ( Fig. 1e ) as well as the complex of FRQ with a purified glutathion- S -transferase (GST)-tagged FRH ( Supplementary Fig. 1e ) contained apparently stoichiometric amounts of both proteins, supporting that the native complex is composed of a dimer or even trimer of FRQ–FRH protomers. It has been suggested that the FFC facilitates rhythmic turnover of frq RNA [14] . The mutant frq 9 allele expresses full-length RNA but, due to a frameshift mutation, it encodes a truncated FRQ 9 protein that does not associate with FRH [14] . We inhibited transcription in WT and frq 9 strains with thiolutin [14] and found that the turnover kinetics of frq and frq 9 RNA was similar ( Supplementary Fig. 2a ), suggesting that the FFC may not regulate turnover of frq RNA. To assess the function of the ATPase of FRH in the circadian clock, we mutated the Walker A and DEXH box motifs ( Supplementary Fig. 2b ), elements required for ATP binding and hydrolysis, respectively [21] , [22] . As FRH is essential for the viability of Neurospora [7] , we expressed mutant and WT versions of FLAG-tagged FRH in an frh + background. The FLAG-tagged FRH versions comprised ~20% of the total FRH ( Fig. 2a ) and did neither affect FRQ expression levels nor circadian rhythms ( Supplementary Fig. 2c ). FLAG-immunoprecipitation (FLAG-IP) revealed that substantially less FRQ was in complex with the mutant FLAG FRH versions than with the WT FLAG FRH ( Fig. 2b ). When protein synthesis was inhibited with cycloheximide, FRQ in complex with the FLAG FRH (followed by FLAG-IP) was degraded with a half-time of 3.5 h ( Fig. 2c ), which corresponds to the previously reported degradation kinetics of FRQ [6] , [23] . FRQ in complex with Walker A and DEAD box mutants of FLAG FRH was degraded significantly faster ( Fig. 2c ). Thus, the turnover of FRQ is directly or indirectly modulated by ATP binding and hydrolysis of FRH. 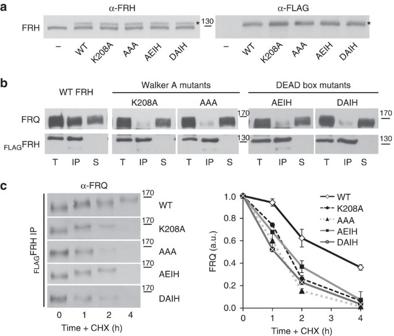Figure 2: Characterization of the FRQ–FRH interaction. (a) Western blot analysis of the indicated FLAG-tagged FRH versions expressed in afrh+background. WT:FLAGFRH; K208A and AAA: Walker A box mutants; AEIH and DAIH: DEAD box mutants. FRH antibody and FLAG antibody was used for decoration in the left and right panel, respectively. Asterisks indicate FLAG-tagged FRH. (b) FRQ does not stably accumulate in complex with ATPase and DEAD box mutants of FRH. Co-IP of FRQ withFLAGFRH versions pulled down with M2 FLAG Sepharose is shown. Protein extracts of light-grown cultures expressingWTand mutant versions of FLAG-tagged FRH were used. Western blots of the total protein extract (T), the immunoprecipitate (IP) and the supernatant (S) were decorated with FRQ antibody (upper panels) and FLAG antibody (lower panels). (c) Turnover kinetics of FRQ in complex with FLAG–FRH versions. Light-grown cultures were incubated with cycloheximide (CHX). Samples were harvested at the indicated time points and the indicatedFLAGFRH versions were immunoprecipitated (FLAG-IP). Immunoprecipitates of mutant FRH versions are five-fold overrepresented. Co-IP of FRQ was detected by western blotting (left panel) and quantified by densitometry (right panel). FRQ levels at time 0 were set equal to 1 (a.u., arbitrary units). Error bars indicate s.d. (n=3). Figure 2: Characterization of the FRQ–FRH interaction. ( a ) Western blot analysis of the indicated FLAG-tagged FRH versions expressed in a frh + background. WT: FLAG FRH; K208A and AAA: Walker A box mutants; AEIH and DAIH: DEAD box mutants. FRH antibody and FLAG antibody was used for decoration in the left and right panel, respectively. Asterisks indicate FLAG-tagged FRH. ( b ) FRQ does not stably accumulate in complex with ATPase and DEAD box mutants of FRH. Co-IP of FRQ with FLAG FRH versions pulled down with M2 FLAG Sepharose is shown. Protein extracts of light-grown cultures expressing WT and mutant versions of FLAG-tagged FRH were used. Western blots of the total protein extract (T), the immunoprecipitate (IP) and the supernatant (S) were decorated with FRQ antibody (upper panels) and FLAG antibody (lower panels). ( c ) Turnover kinetics of FRQ in complex with FLAG–FRH versions. Light-grown cultures were incubated with cycloheximide (CHX). Samples were harvested at the indicated time points and the indicated FLAG FRH versions were immunoprecipitated (FLAG-IP). Immunoprecipitates of mutant FRH versions are five-fold overrepresented. Co-IP of FRQ was detected by western blotting (left panel) and quantified by densitometry (right panel). FRQ levels at time 0 were set equal to 1 (a.u., arbitrary units). Error bars indicate s.d. ( n =3). Full size image Expression and analysis of Neurospora clock proteins in yeast We expressed FRQ, FRH and CK1a in S. cerevisiae to study their interaction and the phosphorylation of FRQ independent of the essential functions of CK1a and FRH in Neurospora . When FRQ was expressed in the absence of FRH and CK1a, it accumulated at a low level and in hypophosphorylated form ( Fig. 3a ). Thus, yeast kinases do not support hyperphosphorylation of FRQ (we define hypo- and hyperphosphorylation operationally by small and large shifts, respectively, in the electrophoretic mobility of FRQ). Co-expression with FRH resulted in elevated expression levels of FRQ, and its phosphorylation state was slightly lower than in the absence of FRH ( Fig. 3a and Supplementary Fig. 3a ). This demonstrates that FRH stabilizes FRQ and suppresses low-level phosphorylation of FRQ by yeast kinases. Mtr4p, the yeast orthologue of FRH [7] , does not interact with FRQ ( Supplementary Fig. 3b ) and does not substitute for the stabilizing function of FRH. When co-expressed with CK1a, FRQ accumulated at a low level and in a hyperphosphorylated form ( Fig. 3a ). Finally, when co-expressed with both, CK1a and FRH, steady-state levels of FRQ were elevated and it was heterogeneously phosphorylated, reminiscent to the steady state of FRQ in light-grown Neurospora ( Fig. 3a and Supplementary Fig. 3c ). The data show that FRH attenuates CK1a-dependent hyperphosphorylation of FRQ. 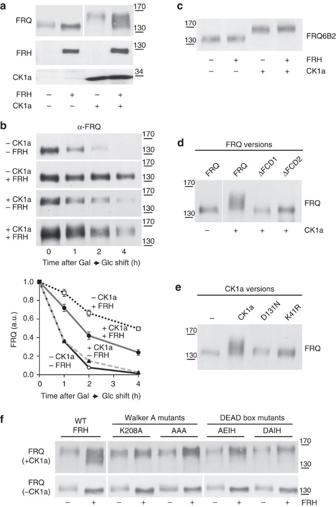Figure 3: Expression and analysis ofNeurosporaclock proteins in yeast. (a) FRH stabilizes FRQ and attenuates its CK1a-dependent hyperphosphorylation. FRQ, FRH and CK1a were expressed inS. cerevisiaeand expression levels and phosphorylation state were analysed by western blot. (b) The degradation kinetics of FRQ is dependent on FRH and CK1a.S. cerevisiaestrains expressing FRQ under control of the GAL1 promoter together with CK1a and FRH when indicated were shifted from galactose to glucose containing medium. Samples were harvested at the indicated time points and analysed by immunoblotting with FRQ antibodies (upper panel). FRQ levels were quantified by densitometry (lower panel). Error bars indicate s.d. (n=3). It should be noted that the apparent degradation kinetics includes dilution of FRQ because of growth of the yeast cells. (c) Expression levels in yeast and phosphorylation state of FRQ6B2 (ref.14) are independent of FRH. FRQ6B2 is a mutant that does not interact with FRH. (d) CK1a-dependent phosphorylation of FRQ is dependent on the CK1a interaction domains FCD1 and FCD2 of FRQ. Western blot analysis of the phosphorylation state of indicated FRQ versions expressed in yeast. Co-expression of CK1a is indicated. (e) The phosphorylation state of FRQ is dependent on expression of catalytically active CK1a. FRQ was co-expressed in yeast with active CK1a and with the catalytically inactive versions D131N and K41R as indicated. (f) ATP binding and hydrolysis by FRH regulates CK1a-dependent hyperphosphorylation of FRQ but the ATPase activity of FRH is not required for the stabilization of FRQ. FRQ was expressed without and with FRH versions as indicated. Upper panel: CK1a was co-expressed. Lower panel: No co-expression of CK1a. FRQ expression level and phosphorylation state were analysed by western blotting. Hyper- and hypophosphorylated FRQ accumulated in the presence (upper panel) and absence (lower panel) of CK1a, respectively. Hyperphosphorylation was attenuated byWTFRH but not by the FRH mutants. Figure 3: Expression and analysis of Neurospora clock proteins in yeast. ( a ) FRH stabilizes FRQ and attenuates its CK1a-dependent hyperphosphorylation. FRQ, FRH and CK1a were expressed in S. cerevisiae and expression levels and phosphorylation state were analysed by western blot. ( b ) The degradation kinetics of FRQ is dependent on FRH and CK1a. S. cerevisiae strains expressing FRQ under control of the GAL1 promoter together with CK1a and FRH when indicated were shifted from galactose to glucose containing medium. Samples were harvested at the indicated time points and analysed by immunoblotting with FRQ antibodies (upper panel). FRQ levels were quantified by densitometry (lower panel). Error bars indicate s.d. ( n =3). It should be noted that the apparent degradation kinetics includes dilution of FRQ because of growth of the yeast cells. ( c ) Expression levels in yeast and phosphorylation state of FRQ6B2 (ref. 14 ) are independent of FRH. FRQ6B2 is a mutant that does not interact with FRH. ( d ) CK1a-dependent phosphorylation of FRQ is dependent on the CK1a interaction domains FCD1 and FCD2 of FRQ. Western blot analysis of the phosphorylation state of indicated FRQ versions expressed in yeast. Co-expression of CK1a is indicated. ( e ) The phosphorylation state of FRQ is dependent on expression of catalytically active CK1a. FRQ was co-expressed in yeast with active CK1a and with the catalytically inactive versions D131N and K41R as indicated. ( f ) ATP binding and hydrolysis by FRH regulates CK1a-dependent hyperphosphorylation of FRQ but the ATPase activity of FRH is not required for the stabilization of FRQ. FRQ was expressed without and with FRH versions as indicated. Upper panel: CK1a was co-expressed. Lower panel: No co-expression of CK1a. FRQ expression level and phosphorylation state were analysed by western blotting. Hyper- and hypophosphorylated FRQ accumulated in the presence (upper panel) and absence (lower panel) of CK1a, respectively. Hyperphosphorylation was attenuated by WT FRH but not by the FRH mutants. Full size image FRQ is an intrinsically unfolded protein [23] . We asked whether FRH and CK1a affect the turnover of FRQ in yeast. The degradation kinetics of FRQ in the absence of FRH was fast ( t 1/2 ~0.5 h), regardless of whether CK1a was present or absent ( Fig. 3b ). Thus, CK1a-dependent hyperphosphorylation of FRQ is not rate determining for degradation of FRQ in the absence of FRH. In the presence of FRH but absence of CK1a, FRQ was rather stable ( t 1/2 ~4 h) ( Fig. 3b ), confirming that FRH stabilizes FRQ [18] . Finally, in the presence of FRH and CK1a, FRQ displayed intermediate stability ( t 1/2 ~1.5 h) ( Fig. 3b ). Together, the data suggest that the turnover of FRQ in complex with FRH is regulated by CK1a-dependent hyperphosphorylation. The FRQ6B2 mutant, in which amino-acid residues 774–776 were exchanged by alanyl residues, is compromised in complex formation with FRH [15] . When expressed in S. cerevisiae, FRQ6B2 was hypophosphorylated in the absence of CK1a and hyperphosphorylated in the presence of CK1a ( Fig. 3c ). Co-expression of FRH did neither support accumulation of elevated levels of FRQ6B2 nor attenuate its CK1a-dependent hyperphosphorylation. Thus, association with FRH is required for the stabilization of FRQ and for the modulation of its CK1a-dependent phosphorylation state. The interaction of FRQ with CK1a is dependent on FCD1 and FCD2, two short putative coiled-coil motifs that interact with each other over a long distance to form directly or indirectly a binding site for CK1a [23] . When FRQΔFCD1 and FRQΔFCD2, deletion mutants lacking one of these motifs, were co-expressed with CK1a, the mutant FRQ versions remained hypophosphorylated ( Fig. 3d ). Thus, despite the expression of high levels of CK1a in yeast, binding of CK1a to FRQ is required for efficient hyperphosphorylation. We then co-expressed FRQ with predicted catalytically inactive versions of CK1a. The mutant kinases CK1aK41R and CK1aD131N [24] , [25] associated with FRQ ( Supplementary Fig. 3d ) but did not support hyperphosphorylation of FRQ ( Fig. 3e ), demonstrating that CK1a does not simply fulfil a structural role in the complex. We then co-expressed FRQ with Walker A and DEXH box mutants of FRH, respectively. The mutant and WT versions of FRH associated with FRQ ( Supplementary Fig. 3e ). The mutant versions of FRH stabilized FRQ in the absence and presence of CK1a but did not attenuate hyperphosphorylation of FRQ in the presence of CK1a ( Fig. 3f ). Expression levels of CK1a were similar in all strains, indicating that the attenuated phosphorylation of FRQ in the presence of WT FRH was not limited by CK1a ( Supplementary Fig. 3f ). Thus, the association with catalytically inactive FRH is sufficient for the protection of FRQ against degradation, while ATP binding and hydrolysis by FRH regulates CK1a-dependent hyperphosphorylation of FRQ. Phosphorylation of FRQ in cell-free extracts We next characterized phosphorylation of FRQ by recombinant CK1a in a cell-free system [26] . Light-grown Neurospora expresses high levels of heterogeneously phosphorylated FRQ. When a native protein extract (cytosol) of such mycelia was incubated with recombinant His6 CK1a at 30 °C, the endogenous FRQ was specifically hyperphosphorylated in a concentration-dependent manner ( Fig. 4a ). Efficient hyperphosphorylation of FRQ was observed at rather high His6 CK1a concentration when the recombinant kinase was present in huge molar excess over FRQ. Notably, endogenous CK1a present in the Neurospora cytosol did not support hyperphosphorylation at 30 °C, although FRQ can be efficiently immunoprecipitated in a complex with endogenous CK1a at 4 °C (refs 6 , 27 ). To characterize the temperature-dependent-binding equilibrium of CK1a and FRQ, we analysed their interaction by immunoprecipitation at 4 and 30 °C ( Fig. 4b ). FRQ co-immunoprecipitated efficiently with CK1a at 4 °C, whereas the interaction was less efficient at 30 °C, indicating that the dissociation of the CK1a–FRQ interaction is rather fast at physiological temperatures. FLAG-tagged CK1a displayed similar temperature-dependent binding to FRQ ( Supplementary Fig. 4a ). To analyse the temperature dependence of the activity of CK1a, we used β-casein as a substrate. As expected, the catalytic activity of recombinant His6 CK1a was higher at 30 °C than at 4 °C ( Fig. 4c ). We then prepared Neurospora cytosol from light-grown cultures, containing heterogeneously phosphorylated FRQ or cytosol from light-induced cultures containing hypophosphorylated FRQ. The cytosols were incubated overnight in the presence of ATP without and with additional recombinant His6 CK1a at 4 °C to stabilize the interaction of CK1a with FRQ. Under these conditions, heterogeneously as well as hypophosphorylated FRQ was efficiently hyperphosphorylated in the presence and also in the absence of additional recombinant His6 CK1a ( Fig. 4d , left panel and Supplementary Fig. 4b ), indicating that the concentration of endogenous CK1a was sufficient for hyperphosphorylation of FRQ under conditions that favour binding of the kinase to FRQ. We then prepared cytosol from strains expressing FRQ versions lacking the CK1a interaction domains FCD1 and FCD2. When these cytosols were incubated with ATP at 4 °C, the FRQΔFCD versions were neither hyperphosphorylated by endogenous CK1a nor by high amounts of recombinant His6 CK1a ( Fig. 4d ). The data demonstrate that FRQ is hyperphosphorylated in cis by bound CK1a. The reaction is limited by the binding equilibrium of CK1a and FRQ (strengthened at 4 °C) rather than by the catalytic activity of CK1a (higher at 30 °C). Free His6 CK1a, even in huge molar excess and in high concentration, does not support efficient phosphorylation, indicating that FRQ is a rather poor substrate for free CK1a. 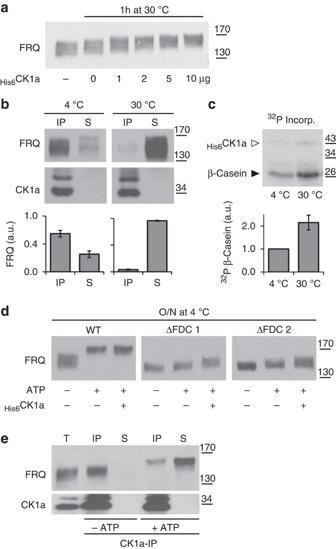Figure 4: Phosphorylation of FRQ in cell-free extracts. (a) CK1a-dependent hyperphosphorylation of FRQ in a cell-free system. Native protein extract of light-grownNeurosporaexpressing heterogeneously phosphorylated FRQ (lane 1) was incubated for 1 h at 30 °C with the indicated amounts of recombinantHis6CK1a. The phosphorylation state of FRQ was dependent on theHis6CK1a concentration. (b) Temperature-dependent interaction of CK1a and FRQ. Native cytosol was prepared fromWTand CK1a was immunoprecipitated at 4 and 30 °C. Aliquots of IP and supernatant (S) were analysed by western blot. FRQ and CK1a signals were quantified by densitometry. Error bars indicate s.d. (n=3). FRQ co-immunoprecipitated with higher efficiency at 4 °C than at 30 °C. (c) Temperature dependence ofHis6CK1a activity. RecombinantHis6CK1a and β-casein were incubated with γ-32P ATP for 1 h at 4 and 30 °C, respectively. Phosphorylation of β-casein and autophosphorylation of CK1a was detected by autoradiography and quantified. Error bars indicate s.d. (n=3). (d) Hyperphosphorylation of FRQin vitrois dependent on CK1a interaction domains (FCDs) even at highHis6CK1a concentration. Protein extracts from cultures expressingWTFRQ and FRQΔFCD1 and FRQΔFCD2, respectively, were incubated overnight at 4 °C in the absence or presence of ATP and purified recombinantHis6CK1a as indicated. The phosphorylation state of FRQ was analysed by immunoblotting. (e) Hyperphosphorylation of FRQ reduces its affinity for CK1a. CK1a was immunoprecipitated overnight at 4 °C fromWTcytosol (containing endogenous FRQ and CK1a) in the absence or presence of ATP. Without ATP, FRQ remained heterogeneously phosphorylated and co-immunoprecipitated efficiently with CK1a. With ATP, FRQ was hyperphosphorylated and its association with CK1a was reduced. Total protein extract before incubation (T), the IP and the supernatant (S) are shown. A three-fold excess of IP and S were loaded with respect to T. Figure 4: Phosphorylation of FRQ in cell-free extracts. ( a ) CK1a-dependent hyperphosphorylation of FRQ in a cell-free system. Native protein extract of light-grown Neurospora expressing heterogeneously phosphorylated FRQ (lane 1) was incubated for 1 h at 30 °C with the indicated amounts of recombinant His6 CK1a. The phosphorylation state of FRQ was dependent on the His6 CK1a concentration. ( b ) Temperature-dependent interaction of CK1a and FRQ. Native cytosol was prepared from WT and CK1a was immunoprecipitated at 4 and 30 °C. Aliquots of IP and supernatant (S) were analysed by western blot. FRQ and CK1a signals were quantified by densitometry. Error bars indicate s.d. ( n =3). FRQ co-immunoprecipitated with higher efficiency at 4 °C than at 30 °C. ( c ) Temperature dependence of His6 CK1a activity. Recombinant His6 CK1a and β-casein were incubated with γ- 32 P ATP for 1 h at 4 and 30 °C, respectively. Phosphorylation of β-casein and autophosphorylation of CK1a was detected by autoradiography and quantified. Error bars indicate s.d. ( n =3). ( d ) Hyperphosphorylation of FRQ in vitro is dependent on CK1a interaction domains (FCDs) even at high His6 CK1a concentration. Protein extracts from cultures expressing WT FRQ and FRQΔFCD1 and FRQΔFCD2, respectively, were incubated overnight at 4 °C in the absence or presence of ATP and purified recombinant His6 CK1a as indicated. The phosphorylation state of FRQ was analysed by immunoblotting. ( e ) Hyperphosphorylation of FRQ reduces its affinity for CK1a. CK1a was immunoprecipitated overnight at 4 °C from WT cytosol (containing endogenous FRQ and CK1a) in the absence or presence of ATP. Without ATP, FRQ remained heterogeneously phosphorylated and co-immunoprecipitated efficiently with CK1a. With ATP, FRQ was hyperphosphorylated and its association with CK1a was reduced. Total protein extract before incubation (T), the IP and the supernatant (S) are shown. A three-fold excess of IP and S were loaded with respect to T. Full size image We then asked whether the phosphorylation state of FRQ affects its interaction with CK1a. Neurospora cytosol was incubated overnight without and with ATP, and CK1a was then immunodepleted ( Fig. 4e ). In the absence of ATP, FRQ remained heterogeneously phosphorylated and co-immunoprecipitated efficiently with CK1a. In the presence of ATP, FRQ was hyperphosphorylated and its co-immunoprecipitation with CK1a was severely reduced. The data indicate that binding of CK1a to FRQ is compromised by hyperphosphorylation of FRQ. As FRQ recruits CK1a to phosphorylate and inactivate its transcription activator WCC, the data suggest that the hyperphosphorylation-dependent loss of CK1a functionally inactivates the FFC as a circadian inhibitor, which should relieve the negative feedback in the core oscillator independent of and before the degradation of FRQ. Reconstitution of Neurospora clock protein interactions in vitro To characterize the phosphorylation of FRQ in vitro, we incubated recombinant FRQ with His6 CK1a and ATP at 30 °C. Under these conditions, FRQ was phosphorylated only to a limited extent and not hyperphosphorylated ( Fig. 5a ). Members of the CK1 protein family catalyse de novo phosphorylation of serine and threonine residues in a negatively charged environment and, in addition, phosphate-directed phosphorylation of S/T P X 2/3 S/T motifs that were previously phosphorylated by a priming kinase [28] . To allow priming phosphorylation, we incubated recombinant FRQ at 30 °C with and without purified His6 CK1a in the presence of either cytosol of a Δfrq strain or yeast cytosol ( Fig. 5b ). In the presence of cytosol but in the absence of His6 CK1a, recombinant FRQ was hypophosphorylated, demonstrating that neither Neurospora kinases (including endogenous CK1a) nor yeast kinases supported efficient hyperphosphorylation of recombinant FRQ under these conditions. However, when His6 CK1a was added together with Neurospora or yeast cytosol, FRQ was efficiently hyperphosphorylated ( Fig. 5b ), suggesting that the cytosols supported in promiscuous manner priming phosphorylation of FRQ, which then served as substrate for His6 CK1a. Hyperphosphorylation of FRQ was dependent on the concentration of His6 CK1a, despite molar excess of the kinase over recombinant FRQ ( Supplementary Fig. 5a ), suggesting a limitation of the reaction by the binding equilibrium of His6 CK1a and FRQ. Recombinant FRQ was then incubated with ATP and Δfrq cytosol at 4 and 30 °C to strengthen and weaken, respectively, complex formation of FRQ with the endogenous CK1a present in the Neurospora cytosol ( Fig. 5c ). FRQ was hyperphosphorylated at 4 °C but not at 30 °C, supporting that the reaction was limited by the binding equilibrium of endogenous CK1a to recombinant FRQ. 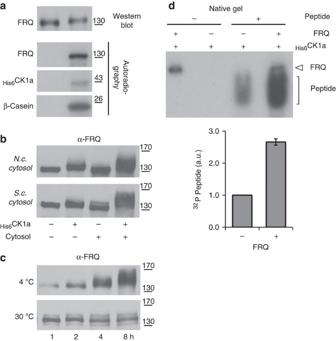Figure 5: Functional interaction of recombinant FRQ and CK1ain vitro. (a)His6CK1a phosphorylates recombinant FRQ only to a limited extend. Purified recombinant FRQ (100 ng) andHis6CK1a (5 μg) were incubated with γ-32P ATP for 1 h at 30 °C. The upper panel shows a western blot analysis of FRQ. The lower panels are autoradiograms showing incorporation of32P into recombinant FRQ,His6CK1a (autophosphorylation) and β-casein (CK1a activity control). (b) Hyperphosphorylation of recombinant FRQ byHis6CK1a is dependent on priming kinases supplied by cytosol ofNeurospora crassa(N.c.) orS. cerevisiae(S.c.). Recombinant FRQ (100 ng) was incubated in the absence or presence ofHis6CK1a (5 μg) with and without cytosol (400 μg) of aN.c. frq10(Δfrq) strain or yeast cytosol when indicated. The samples were incubated 1 h at 30 °C. (c) CK1a present inNeurosporacytosol supports hyperphosphorylation of recombinant FRQ at 4 °C but not at 30 °C. Purified FRQ (100 mg) was incubated withfrq10cytosol for the indicated time periods. (d) CK1a is activated by recruitment to FRQ.His6CK1a (100 ng) was pre-incubated for 30 min at 4 °C with a four-fold molar excess of recombinant FRQ (1 μg) to allow stable complex formation or with 1 μg BSA to balance the total protein content. Subsequently, the phosphopeptide Ac-KRRRALS(pS)VASLdP(Sox)G-NH (2 μg) (Life Technologies) was incubated at 4 °C with γ-32P ATP (25 μM) and with either the preformedHis6CK1a-FRQ complex or the corresponding amount of freeHis6CK1a (+BSA). Reactions were terminated after the indicated time periods and analysed by native-PAGE and autoradiography (upper panel). FRQ and the peptide were phosphorylated. BSA was not phosphorylated and autophosphorylation of CK1a is not visible at the shown exposure. Lower panel: phosphorylation of the peptide was quantified by densitometry. Error bars indicate s.d. (n=3). Figure 5: Functional interaction of recombinant FRQ and CK1a in vitro. ( a ) His6 CK1a phosphorylates recombinant FRQ only to a limited extend. Purified recombinant FRQ (100 ng) and His6 CK1a (5 μg) were incubated with γ- 32 P ATP for 1 h at 30 °C. The upper panel shows a western blot analysis of FRQ. The lower panels are autoradiograms showing incorporation of 32 P into recombinant FRQ, His6 CK1a (autophosphorylation) and β-casein (CK1a activity control). ( b ) Hyperphosphorylation of recombinant FRQ by His6 CK1a is dependent on priming kinases supplied by cytosol of Neurospora crassa ( N.c .) or S. cerevisiae ( S.c. ). Recombinant FRQ (100 ng) was incubated in the absence or presence of His6 CK1a (5 μg) with and without cytosol (400 μg) of a N.c. frq 10 (Δfrq ) strain or yeast cytosol when indicated. The samples were incubated 1 h at 30 °C. ( c ) CK1a present in Neurospora cytosol supports hyperphosphorylation of recombinant FRQ at 4 °C but not at 30 °C. Purified FRQ (100 mg) was incubated with frq 10 cytosol for the indicated time periods. ( d ) CK1a is activated by recruitment to FRQ. His6 CK1a (100 ng) was pre-incubated for 30 min at 4 °C with a four-fold molar excess of recombinant FRQ (1 μg) to allow stable complex formation or with 1 μg BSA to balance the total protein content. Subsequently, the phosphopeptide Ac-KRRRALS(pS)VASLdP(Sox)G-NH (2 μg) (Life Technologies) was incubated at 4 °C with γ- 32 P ATP (25 μM) and with either the preformed His6 CK1a-FRQ complex or the corresponding amount of free His6 CK1a (+BSA). Reactions were terminated after the indicated time periods and analysed by native-PAGE and autoradiography (upper panel). FRQ and the peptide were phosphorylated. BSA was not phosphorylated and autophosphorylation of CK1a is not visible at the shown exposure. Lower panel: phosphorylation of the peptide was quantified by densitometry. Error bars indicate s.d. ( n =3). Full size image We then asked whether CK1a is activated by recruitment to FRQ. To efficiently drive complex formation, CK1a was incubated at 4 °C with an ~four-fold molar excess of recombinant FRQ. Subsequently, we incubated a CK1 phosphopeptide substrate ( Fig. 5d ) or β-casein ( Supplementary Fig. 5b ) at 4 °C with either the preformed His6 CK1a-FRQ complex or with the corresponding amount of free His6 CK1a. Both substrates were more efficiently phosphorylated by the preformed His6 CK1a-FRQ complex than by free His6 CK1a ( Fig. 5d and Supplementary Fig. 5b ). The data suggest that the catalytic site of FRQ-associated CK1a is accessible for substrate in cis and trans . Moreover, CK1a is activated by recruitment to FRQ. In this way, a single molecule of bound CK1a could phosphorylate in cis a large number of sites that are distributed all over the intrinsically disordered polypeptide chain of FRQ and also WCC that is recruited to the FFC [16] , [17] , [29] . Progressive hyperphosphorylation is a hallmark of clock proteins in all eukaryotic model systems and correlates strongly with circadian timing. We show here that FRH, the Neurospora orthologue of the S. cerevisiae RNA helicase MTR4, modulates the slowly progressing phosphorylation of FRQ on a circadian timescale. FRH associates with and stabilizes FRQ in ATP-independent manner, while the ATPase of FRH attenuates the kinetics of CK1a-dependent hyperphosphorylation of FRQ. The regulatory function of FRH in the FRQ complex is independent of its essential RNA helicase activity in the TRAMP complex and exosome pathway, and hence, FRH has two mechanistically distinct functions. In vitro studies with recombinant FRQ and FRH as well as analysis of the Neurospora clock proteins in S. cerevisiae indicate that the FRQ–FRH interaction is tight and is not dependent on ATP, but it is not known whether the ATPase of FRH modulates a transient dissociation–association cycle. We show that hyperphosphorylation of FRQ is dependent on priming kinases and on CK1a. Priming phosphorylation of FRQ is provided by S. cerevisiae , suggesting that the priming kinases are rather promiscuous. In Neurospora , FRQ is phosphorylated by CKII (ref. 30 ), calcium/calmodulin-dependent kinase [31] and protein kinase A [32] . Hence these kinases may, in addition to their putative specific roles, serve as priming kinases. In contrast to priming phosphorylation, subsequent hyperphosphorylation of FRQ is strictly dependent on Neurospora CK1a. The phosphorylation reaction is limited by the FRQ–CK1a-binding equilibrium. Free CK1a is rather inactive and becomes catalytically activated by recruitment to FRQ via FCD1 and FCD2. The FRQ-dependent activation of CK1a did not require FRH. Interestingly, it has recently been shown that CK1ε, a mammalian homologue of CK1a, is activated by recruitment to the human RNA helicase DDX3 to phosphorylate its substrate dishevelled in a wnt/β-catenin signalling complex [33] . Like the FFC, the wnt/β-catenin signalling complex contains a DEAD box helicase, CK1 and substrate. CK1ε is recruited to the complex by DDX3 (the helicase) while CK1a is recruited by FRQ (the substrate). In both systems, CK1, a simple monomeric enzyme, is rather inactive and is activated by site-specific recruitment to a target complex. The co-occurrence of a DEAD box helicase and CK1 in both, the Neurospora clock complex and in the wnt/β-catenin signalling complex [33] may suggest a conserved functional interaction of RNA helicases and CK1 in protein complexes. However, while the ATPase of FRH regulates the activity of CK1a, a putative regulatory function of the conserved ATPase of DDX in the wnt/β-catenin pathway has not been uncovered. How can one CK1a molecule that is bound to a specific site in FRQ facilitate phosphorylation of a large number of sites distributed throughout the polypeptide chain [4] , [5] ? FRQ is an intrinsically unfolded protein [18] , [23] . The few predicted folded segments correspond to the N-terminal coiled-coil domain that facilitates oligomerization of FRQ, the two FCDs in the central portion, which interact with each other via a coiled-coil and the FRH interaction domain in the C-terminal portion of FRQ [7] , [19] , [23] . The remaining portions of FRQ are predicted to be unstructured. These potentially flexible random coils may eventually reach the catalytic site of a CK1a molecule bound to FRQ via the FCDs. A tightly bound, activated CK1a molecule corresponds to a high local kinase concentration, which may further facilitate phosphorylation in cis . It is not known whether the progressive phosphorylation of FRQ is entirely random or follows an obligate (or preferentially) sequential temporal pattern similar to the sequential phosphorylation of certain sites in PERIOD of Drosophila [34] . FRH attenuates the overall phosphorylation kinetics of FRQ. As FRQ is phosphorylated at up to ~100 sites [4] , [5] , the question arises how FRH can modulate the phosphorylation kinetics of FRQ at many different sites. Our data suggest that ATP hydrolysis by FRH may remodel the complex such that the access of CK1a to phosphorylation sites in FRQ is compromised. The ATPase cycle of FRH may thus control the temporal progression of the phosphorylation of FRQ that is crucial for the molecular timing process. Structural and functional analysis of recombinant clock components in vitro will help elucidating the detailed molecular mechanism. Recently, it has been suggested that the ATPase of FRH is not required for the function of the circadian clock [18] . As FRH is essential for the viability of Neurospora , this conclusion was based on co-expression of two FRH alleles, one with a defect in the clock supplying the essential function of FRH, and the other with a defective ATPase. To be conclusive, it is mandatory that FRH does not form a homodimer in its interaction with FRQ dimers, as dimerization of FRH could lead to the formation of a FFC bearing one helicase null FRH and one clock null FRH, thereby allowing for cross-complementation [18] . We show that a monomeric mutant version of FRQ interacts with one molecule of FRH. As WT FRQ is a dimer or a higher oligomer [19] , the complex should contain stoichiometric amounts of FRH unless a specific mechanism would exclude binding of a second FRH molecule. The apparent molecular mass of the WT FFC and the reconstituted FFC (~670 kDa) suggests an assembly of at least two FRQ and two FRH molecules. Recent mass spectrometry analysis suggested that the interaction of FRQ with CK1a decreases in the course of a day by an unknown mechanism [5] . We show here that hyperphosphorylation of FRQ compromises its interaction with CK1a. The FCD1/2 interaction, which is considerably weak, appears to be additionally stabilized by ionic interactions of the positively charged N terminus with the negatively charged middle and C-terminal portions of FRQ [23] . Hence, in the course of a circadian period, CK1a-dependent hyperphosphorylation of the positively charged N terminus may progressively weaken the FCD1/2 coiled-coil shifting of the CK1a–FRQ-binding equilibrium gradually towards dissociation. In the core feedback loop of the Neurospora clock, the FFC complex transiently recruits and inactivates the circadian transcription factor WCC by facilitating its phosphorylation by bound CK1a [29] . The release of CK1a from hyperphosphorylated FRQ will functionally inactivate the FFC before proteolytic degradation of FRQ. Thus, inactivation of FRQ might be functionally more important for the circadian feedback loop than protein degradation. Degradation of FRQ might be required to maintain homeostasis, as accumulation of high levels of inactive FRQ could feedback (for example, via dephosphorylation) on the steady-state concentrations of active FRQ. It is not known whether clock proteins in other eukaryotic systems are regulated in similar manner. In the circadian clock of cyanobacteria KaiA and B proteins regulate independently of protein turnover autophosphorylation/dephosphorylation cycles and assembly state of KaiC hexamers [35] . KaiC oscillator contains two ATP-binding domains, CI and CII. The CII domain has autokinase/phosphatase activity crucial for the circadian timing process [36] , [37] , and the slow ATPase of CI may act as an input-independent timer [38] . Regulation of FRQ by the two ATPases, CK1a and FRH, could be functionally similar to the regulation of KaiC by its CI and CII domains. In summary, FRQ, the FRH ATPase and the CK1a kinase form a molecular timing device driven by two ATP-dependent processes. Hyperphosphorylation of FRQ is dependent on activated CK1a bound to FRQ. The ATPase cycle of FRH attenuates the phosphorylation kinetics on a circadian timescale leading to a progressive inactivation of the circadian inhibitor complex via dissociation of CK1a. It is tempting to speculate that DEAD box-containing RNA helicases such as FRH could be more general ATPase-driven remodelling machines/modules that may, depending on their recruitment to specific complexes, drive conformational changes in double-stranded RNA structures and protein complexes in mechanistically similar manner. Neurospora strains and culture conditions Neurospora strains that were used in this study (WT, frq10, frq9, FRQΔNLS [20] , ΔFCD1, ΔFCD2 (ref. 23 ), frq + FLAG FRH WT, frq + FLAG FRH Walker A mutants and frq + FLAG FRH DEIH mutants) all carried the ras-1 bd mutation [39] . Conidial suspensions in 1 M sorbitol were prepared from strains grown (5–7 days) on standard solid growth medium (2.2% agar, 0.3% glucose, 0.17% L -arginine, 1 × Vogel’s medium and 0.1% biotin). Standard growth medium for liquid cultures contained 2% glucose, 0.17% L -arginine and 1 × Vogel’s medium. The cultures were grown in constant light at 25 °C for 48 h if not indicated otherwise. Cycloheximide was added at a concentration of 10 μg per ml and thiolutin was added to a final concentration of 12 μg per ml where indicated. The race tube medium contained 2% agar, 0.1% glucose, 0.17% L -arginine, 1 × Vogel’s medium and 0.1% biotin. The race tubes were evaluated by densitometry and the Chrono ll software (T. Roenneberg, Ludwig-Maximilians-Universität Munich). S. cerevisiae culture conditions Yeast cells of the strain DS1-2b (Y2197; MAT, his3-Δ200 leu2-Δ1 trp1-Δ63 ura3-52, kindly provided by the Hurt group/University of Heidelberg Biochemistry Centre) for transformations with the respective vectors were grown in rich YPD medium. Transformation was performed as described previously [40] . Yeast strains were grown in selection medium: synthetic dextrose complete medium or synthetic raffinose complete medium. Synthetic raffinose complete medium was used if a construct containing a galactose promoter was present in a strain. Galactose was added to a final concentration of 1%. Pre-cultures were grown overnight at 30 °C and 120 r.p.m. and used to inoculate new cultures that were grown to OD 600 =0.5 to further proceed with experimental procedures. Plasmid construction The Neurospora vector pMF309 (ref. 41 ) was used as a backbone for ccg-1-flag-frh constructs. A genomic PCR product was inserted as SpeI-EcoRI fragment (primers:F: 5′- actagt atggactacaaagacgatgatgacaaagattacaaggatgacgacgataagg ggcgcgcc atggacgacctctttgaggttttc -3′ and R:5′- tttctttcaacagtctgtatctgtaa gaattc -3′). The Walker A and DEIH motif were changed by site-directed mutagenesis. Plasmids for expression of FRQ and FRH in yeast (generous gift of Hurt group/University of Heidelberg Biochemistry Centre) were based on: 4383-YCp111-P.ADH1-HA-RSA4 and 4045Y-Cp22-P.Gal-GFP-RSA4. PCR product amplified from complementary DNA was inserted into these vectors as NdeI-NotI and AscI-NotI fragments, respectively. CK1a expressing yeast vectors were generated as described previously [23] . Protein analysis Extraction of Neurospora and S. cerevisiae native protein: Tissue/cells were ground in the presence of liquid nitrogen using a pre-cooled pestle and mortar. The powder was suspended in extraction buffer (50 mM HEPES/KOH (pH 7.4), 137 mM NaCl, 10% (v/v) glycerol, 5 mM EDTA containing 1 mM phenylmethylsulfonylfluoride (PMSF), 5 μg ml −1 leupeptin and 5 μg ml −1 pepstatin A) [29] . Protein concentrations were determined by NanoDrop (PeqLab). Four-hundred micrograms of N . crassa and 100 μg of S. cerevisiae extract were analysed by SDS-PAGE and transferred to a nitrocellulose membrane (GE Healthcare; 0.45 μm, 10 × 150 cm) in 150 mM glycine, 20 mM Tris, 20% (v/v) methanol and 0.08% (w/v) SDS at 200 mA for 2.5 h. The membrane was blocked with TBS and 5% milk (pH 7.4) before incubation with antibodies [6] , [29] . Antibodies against FRQ were used 1:20 diluted in 5% milk and CK1a antibodies at a dilution of 1:500 in 5% milk [6] , [23] . An FRH (1:350 in 5% milk) antibody was raised in rabbits against a peptide corresponding to amino-acid residues 2–18 (Pineda, Berlin). The MTR4 (1:20,000 in 5% milk) antibody was a generous gift of David Tollervey, Edinburgh. Enhanced chemiluminescence signals were detected with X-ray films (Fuji). Several series of exposures were generated and quantified by using the ImageJ software (Rasband, W.S., ImageJ, U. S. National Institutes of Health). Uncropped scans of the most important western blots are shown in Supplementary Fig. 6 . Preparation of yeast denaturing extracts: a volume corresponding to 1.0 OD 600 was removed from exponentially growing cells. Cells were pelleted (3 min at 3,600 r.p.m.) and washed in 1 ml water. Cells were resuspended in 150 μl denaturing extraction buffer (1.85 M NaOH, 7.5% β-mercaptoethanol; freshly prepared) and placed on ice for 10 min. TCA (55%; 150 μl) was added and the mixture was incubated for 10 min on ice. Proteins were precipitated for 10 min at 14,000 g at 4 °C. The pellet was resuspended in 40 μl 0.1 M NaOH and 14 μl 4 × Laemmli sample buffer and incubated at 95 °C for 5 min. Aliquots corresponding to 0.5 OD 600 of cells were analysed by SDS-PAGE [42] . All experiments and western blots were performed at least three times and one representative example is shown. Purification of recombinant proteins Recombinant His-tagged CK1a was purified from E. coli: A pre-culture was grown in LB medium containing ampicillin (100 ng μl −1 ) at 37 °C overnight. The pre-culture was then diluted 1:100 and grown at 37 °C to 0.3 OD 600 , then temperature was lowered to 18 °C. The culture was induced with 0.1 mM IPTG overnight and harvested at 4,000 r.p.m. for 20 min. Following steps were performed at 4 °C. His 6 -tagged kinase was isolated using standard Qiagen protocol for pQE30 vectors (QIA expressionist) with the following changes: the isolation of the His 6 -tagged kinase was done in a cold room using gravity or a pump with max 0.5 ml min −1 flow rate. Elution was performed in three steps with 1 ml elution buffer and 1 min incubation between each step. The samples were immediately re-buffered into Neurospora protein extraction buffer (without glycerol) using PD-10 columns (GE Healthcare). Glycerol was added after re-buffering [26] ). FRH (residues 1–1,106) and FRHΔN (residues 116–1,106) were expressed with an N-terminal His 6 -GST-tag followed by a TEV cleavage site in E. coli BL21(DE3) cells. Proteins were purified using a Ni-nitrilotriacetate (NTA) affinity step followed by TEV cleavage and heparin Sepharose chromatography (GE Healthcare). Size-exclusion chromatography was performed (Superdex 200, GE Healthcare) in 20 mM HEPES pH 7.5, 150 mM NaCl and 2 mM DTT for final purification. FRQ (residues 1–989) was expressed with a N-terminal His 6 -Z-tag [43] followed by a TEV cleavage site in E. coli BL21(DE3) cells. FRQ was purified using a NTA affinity step followed by ion exchange. After ion exchange, the tag was removed by TEV cleavage. The uncleaved fusion protein and the TEV protease were removed by a second NTA affinity step. Size-exclusion chromatography was performed (Superdex 200, GE Healthcare) in 20 mM HEPES, pH 7.5, 250 mM NaCl, 10% glycerol and 2 mM DTT for final purification [13] . Gel filtration Neurospora extracts (10–15 mg) or recombinant clock proteins (5 mg) were loaded (<0.25 ml) on a Superose 6 gel filtration column. Chromatography was performed at 4 °C at a flow rate of 0.5 ml min −1 and fractions of 0.5 ml were collected. In vitro phosphorylation assay The phosphorylation reaction contained 50 mM HEPES/KOH, pH 7.4, 150 mM NaCl, 10 mM MgCl 2 , 10 mM ATP, leupeptin (2 μg per ml), pepstatin A (2 μg per ml), PMSF (1 mM), and PhosStop phosphatase inhibitor cocktail (Roche). Protein extract (400 μg) was incubated with or without recombinant clock proteins (100 ng FRQ, 5 μg 6HIS -CK1a, if not indicated otherwise) in a final volume of 60 μl at 4 or 30 °C. Laemmli sample (4 × ; 18 μl) buffer was added, followed by a 5-min incubation at 95 °C. Aliquots were analysed by SDS gel electrophoresis followed by western Blot analysis with FRQ antibody. Co-immunoprecipitation CK1a IPs were performed as described previously [23] . Affinity-purified FRH antibody was bound to 30 μl protein A Sepharose CL-4B beads (GE Healthcare) for 2 h at room temperature. The beads were washed twice with PBS containing protease and phosphatase (PhosStop, Roche) inhibitors. Cell lysate (5 mg) prepared in PEX buffer was added to the beads. The reaction was filled up with PBS to 500 μl. The mixture was incubated overnight at 4 °C if not indicated otherwise. The beads were washed two times with PBS and the bound protein was eluted in 2 × Laemmli sample buffer for 5 min at 95 °C. For IP of proteins with a FLAG-tag, 30 μl M2 FLAG Sepharose (Sigma) was used. GST pull-down experiment GST–FRH (110 pmol) was incubated with 55, 110 or 220 pmol of FRQ in 500 μl binding buffer (20 mM HEPES/NaOH, 150 mM NaCl, 5% glycerol and 2 mM DTT, pH 7.5) for 2 h on ice. After addition of glutathione beads, the samples were incubated for 2 h at 4 °C, washed three times with 500 μl binding buffer and eluted with 20 mM HEPES/NaOH, 150 mM NaCl, 5% glycerol and 25 mM GSH, pH 7.5. The eluted proteins were analysed by SDS-PAGE. Quantitative real-time PCR Total mRNA from ground frozen mycelia was prepared using peqGOLD TriFAST (PeqLab, Germany) and reverse transcription was performed using the QuantiTect Reverse Transcription Kit (Qiagen, Germany) following the manufacturer’s instructions. Transcript levels were analysed by quantitative real-time PCR (RT-PCR) as described previously [23] . Sequences of primers and probes used for RT–PCR were: frq : F: 5′-ttgtaatgaaaggtgtccgaaggt-3′; R: 5′-ggaggaagaagcggaaaacg-3′; Probe: 6-FAM 5′-acctcccaatctccgaactcgcctg-3′ (TAMRA); 28s rRNA: F: 5′-cctgttcgagcgtcatttca-3′; R: 5′-agcccgccactgattttg-3′; 6-FAM 5′-ccatcaagctctgcttgcgttggg-3′ (TAMRA). How to cite this article: Lauinger, L. et al. The RNA helicase FRH is an ATP-dependent regulator of CK1a in the circadian clock of Neurospora crassa . Nat. Commun. 5:3598 doi: 10.1038/ncomms4598 (2014).